Selective inhibition of BET bromodomain epigenetic signalling interferes with the bone-associated tumour vicious cycle The vicious cycle established between bone-associated tumours and bone resorption is the central problem with therapeutic strategies against primary bone tumours and bone metastasis. Here we report data to support inhibition of BET bromodomain proteins as a promising therapeutic strategy that target simultaneously the three partners of the vicious cycle. Treatment with JQ1, a BET bromodomain inhibitor, reduces cell viability of osteosarcoma cells and inhibits osteoblastic differentiation both in vitro and in vivo . These effects are associated with transcriptional silencing of MYC and RUNX2 , resulting from the depletion of BRD4 from their respective loci. Moreover, JQ1 also inhibits osteoclast differentiation by interfering with BRD4-dependent RANKL activation of NFATC1 transcription. Collectively, our data indicate that JQ1 is a potent inhibitor of osteoblast and osteoclast differentiation as well as bone tumour development. Bone malignancies can be divided into two classes, primary and secondary bone tumours. Secondary bone tumours arise from disseminated tumour cells that originate from distant primary sites, most commonly from breast, prostate and lung cancers, which subsequently give rise to metastatic development in the bone [1] . Malignant primary bone tumours are rare pathologies, with osteosarcoma being the most frequent type in children and young adults and have a poor prognosis owing to its propensity to metastasize. Osteosarcoma is defined as a malignant tumour of mesenchymal cells and its diagnosis is based on histopathological features characterized by the direct formation of abnormal osteoid and/or woven bone [2] . Current therapeutic regimens for osteosarcoma include neoadjuvant and adjuvant chemotherapy combined with tumour resection [3] . While survival rate can reach 70% at 5 years in the best series, survival rate is significantly reduced to only 30% when pulmonary metastases are detected at the time of diagnosis. Thus, the overall clinical outcome remains poor despite treatment advances, which underscores the need to identify novel therapeutic strategies for osteosarcoma. The vicious cycle established between osteoclasts (OCs), bone stromal cells/osteoblasts (OBs) and cancer cells is the driving force of osteolytic lesions during progression of primary bone tumours [4] , [5] , [6] . Histological analyses of osteolytic primary and secondary bone tumours reveal that the bone destruction is mediated by OCs rather than the tumour cells themselves. The tumour cells modify the bone microenvironment and promote the recruitment of OC progenitors by secreting osteoclastic-activating factors such as interleukin (IL)6, tumour necrosis factor-α, IL1 and parathyroid hormone-related protein. The OCs, in turn, resorb bone tissue and release from the bone matrix growth factors that stimulate the proliferation of tumour cells [6] . A key pathway implicated in OC activation is the receptor activator of nuclear factor kappaB (NFkB) and its ligand (RANK/RANKL), which induces the expression of nuclear factor of activated T cells, cytoplasmic 1 (NFATC1), a master transcription factor of OC differentiation and one of its downstream effectors like matrix metallopeptidase 9 (MMP9). Given that the interplay between tumour growth and bone resorption is the basis of the vicious cycle of osteosarcoma, a potential therapeutic strategy is to disrupt this cycle by targeting OC and OB differentiation as well as tumour cell proliferation. Several genes have been identified as drivers of osteosarcoma development. c-MYC (hereafter referred as MYC ) is one of the most highly amplified oncogenes in cancer. It encodes an evolutionarily conserved basic helix-loop-helix leucine zipper transcription factor that is commonly deregulated in numerous types of human malignancies. Owing to a large number of direct transcriptional targets and the resulting activation of many transcriptional and signalling networks, amplification of MYC results in pleiotropic effects on cancer cell survival, proliferation, metastasis and angiogenesis [7] . Genomic amplification at 8q24 and overexpression of MYC has been observed in osteosarcoma [8] , [9] , [10] . Moreover, MYC overexpression in a Ink4/Arf(−/−) context was not only sufficient to transform bone marrow stromal cells but also led to osteosarcoma development [11] . In addition, RUNX2 , a key transcription factor in OB differentiation, appears to be a potential oncogenic driver in osteosarcoma, depending on its expression level and cellular context [12] , [13] , [14] , [15] . Indeed, short interfering RNA (siRNA) knockdown of RUNX2 in U2OS osteosarcoma cells was shown to inhibit cell growth, while overexpression of RUNX2 in T-cell lymphoma synergized with MYC to promote survival and proliferation of cancer cells [13] , [16] . Thus, inhibition of MYC and RUNX2 transcriptional network may be of clinical relevance in osteosarcoma. Histone modifications are of critical importance for the maintenance of the transcription programme of both normal and tumour cells. Post-translational covalent modifications of the histone amino-terminal tail influence chromatin structure and the accessibility of DNA to transcriptional machinery. The bromodomain and extra-terminal domain (BET) protein family (BRD2, BRD3, BRD4 and BRDT) is an important class of ‘epigenetic reader proteins’, which function to recognize the N -acetylation of lysine residues on histone tails [17] . Bromodomain-containing proteins act as a scaffold for molecular complexes at recognized histones’ sites to regulate chromatin accessibility to transcription factors and RNA polymerase [18] . Very recently, BRD4 has been identified as a potent therapeutic target in acute myeloid leukaemia [19] , [20] . Moreover, the BET bromodomain proteins have been shown to regulate the expression of MYC in different tumour types [19] , [20] , [21] , [22] , [23] , [24] , [25] . Several studies have tested the pharmacologic inhibition of bromodomains using JQ1, a thienotriazolo-1,4-diazapine that binds selectively to the acetyl-lysine-binding pocket of the BET bromodomain proteins, inhibiting only BRD2, BRD3, BRD4 and BRDT among the 47 bromodomain proteins with a prevalent affinity for BRD4 (ref. 26 ). Pharmacologic inhibition of bromodomains leads to selective alterations in gene expression most probably owing to the disruption of strong enhancer-mediated transcription at oncogenic loci, such as those bound by MYC . Indeed, gene set enrichment analysis indicates that one of the most deregulated network is the MYC transcriptome [22] . Furthermore, JQ1 treatment resulted in a reduction of MYC expression as well as induced cell death in multiple myeloma, leukaemia and lymphoma both in vitro and in vivo [20] , [21] . In this study, we show that BET bromodomain signalling plays a role in osteosarcoma and that inhibition of this epigenetic recognition pathway suppresses osteosarcoma tumour growth both in vitro and in vivo . We also identify RUNX2 as a new direct transcriptional target of BRD4, linked to the bone-associated tumour context as inhibition of RUNX2 reduced both osteoblastic differentiation and primary bone tumour development. In addition, we show that the unique and selective BET bromodomain inhibitor JQ1 potently represses not only MYC gene expression but also RUNX2 gene expression as well as their transcriptional network in osteosarcoma cell lines and in vivo tumour models. The JQ1-mediated transcriptional silencing of MYC and RUNX2 corresponds with the release of BRD4 from their respective loci, which further supports the direct transcriptional activation of these genes by BRD4 . Finally, we uncover a BRD4-dependent RANKL activation pathway in osteoclastogenesis, which is also inhibited by JQ1 treatment. Taken together, our findings indicate that targeting the BET bromodomain signalling pathway in primary bone cancer can effectively disrupt the vicious cycle through transcriptional repression of oncogenic drivers in osteosarcoma as well as through the inhibition of OB and OC differentiation. Importantly, our work provides a strong clinical rationale for the use of BET bromodomain inhibitors, specifically JQ1, as a therapeutic approach for osteosarcoma. BET bromodomain proteins and MYC overexpression in patients To assess the therapeutic potential of targeting BET bromodomain signalling in osteosarcoma, we first evaluated the messenger RNA expression level in human osteosarcoma patient samples of BRD2, BRD3, BRD4 and BRDT as well as MYC , since it has been associated to the BRD4 inhibition effects [17] , [18] . Compared with normal mesenchymal stem cells (MSCs), 9 out of 14 patients overexpressed both BRD4 and MYC , 11 out of 14 overexpressed BRD2 and MYC and 7 out of 14 overexpressed BRD3 and MYC ( Fig. 1a and Supplementary Fig. 1 ). None of the patients expressed BRDT, which is a tissue-specific protein. This finding suggests that the majority of osteosarcoma patients express the required molecular targets for an inhibition of BET bromodomains epigenetic signalling strategy, which is the minimal rational to make them candidates to this therapy. Moreover, we observed a strong correlation ( P <0.001) between the expression level of BRD4 with MYC , using the Pearson product-moment correlation coefficient ( R 2 ; Fig. 1b ). As the size of our patient cohort was limited, we validated this correlation in a lager cohort of 27 osteosarcoma patients’ biopsy samples obtained by Dr Yamada T from the National Cancer Center of Tokyo (GEO Series GSE14827) [27] . The expression array study confirmed the strong correlation between BRD4 and MYC expression level ( Supplementary Fig. 2 ). 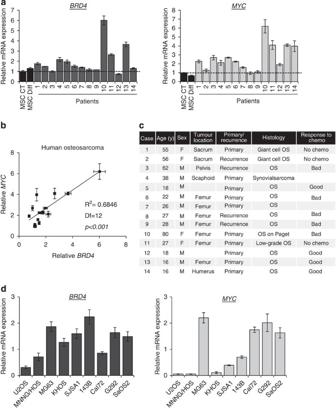Figure 1: Brd4 and MYC messenger RNA levels are overexpressed in osteosarcoma patients. (a) Expression ofBRD4andMYCmRNA levels were evaluated by qRT–PCR in human osteosarcoma biopsies compared with normal cells. (b) Correlation betweenBRD4andMYCexpression in human osteosarcoma specimens, assessed by qRT–PCR and tested by the Pearson product-moment correlation test. (c) Clinical features of osteosarcoma patients. (d) Expression ofBRD4andMYCmRNA levels in human osteosarcoma cell lines, assessed by qRT–PCR. Error bars show s.e.m. forn=3 measurement from representative experiments. Figure 1: Brd4 and MYC messenger RNA levels are overexpressed in osteosarcoma patients. ( a ) Expression of BRD4 and MYC mRNA levels were evaluated by qRT–PCR in human osteosarcoma biopsies compared with normal cells. ( b ) Correlation between BRD4 and MYC expression in human osteosarcoma specimens, assessed by qRT–PCR and tested by the Pearson product-moment correlation test. ( c ) Clinical features of osteosarcoma patients. ( d ) Expression of BRD4 and MYC mRNA levels in human osteosarcoma cell lines, assessed by qRT–PCR. Error bars show s.e.m. for n =3 measurement from representative experiments. Full size image No correlation has been observed between MYC and BRD2 or BRD3 using either our patient tumour samples or the larger Yamada lab cohort. Unfortunately, the sizes of our patient cohort or even the complete Yamada’s patient cohort are not big enough to correlate the clinical outcome of the patient with BRD4 or MYC expression or with age, sex, tumour location, histological origin or response to chemotherapy ( Fig. 1c and Supplementary Fig. 2 ). We then evaluated the BRD2, BRD3, BRD4 and MYC expression level in various patient-derived osteosarcoma cell lines and murine osteosarcoma cell lines. We observed an interesting variability, comparable to our patient cohort, which prompted a more detailed study of BET bromodomain signalling in osteosarcoma ( Fig. 1d and Supplementary Figs 1 and 3 ). Inhibition of BET bromodomain proteins in vitro To evaluate the therapeutic potential of BET bromodomain inhibition in osteosarcoma, we used the pharmacological inhibitor JQ1, a thienotriazolo-1,4-diazapine that binds selectively to the acetyl-lysine-binding pocket of the BET bromodomain protein ( Fig. 2a ) [26] . We first treated a panel of nine genetically defined human osteosarcoma cell lines ( Fig. 2b ) with the BET inhibitor JQ1 to assess its effect on cell viability. A dose-dependent inhibition of cell viability was observed in all cell lines studied. Comparison of the GI 50 of each tumour cell line revealed no significant difference in cell viability sensitivity for MNNG/HOS, KHOS, U2OS and MG63 cell lines as they exhibited a GI 50 between 0.268 and 1.081 μM. In contrast, the others cell lines tested were about 10 times more resistant compared with the first ones, among them, SaOS2 cells with a GI 50 of 6.457 μM ( Fig. 2b ). Then we performed a colony formation assay in the presence or absence of JQ1, which revealed significant differences between the cell lines in terms of their capacity to recover following 2 days of BET inhibitor treatment (1 μM). Indeed, while U2OS and MNNG/HOS exhibited significant reduction in colony formation, MG63 and SaOS2, respectively, exhibited moderate sensitivity or no sensitivity at all to JQ1 treatment ( Fig. 2c,d ). These differences were further confirmed by cell cycle analysis. The proportion of cells in subG 1 (representing dead cells as determined by propidium iodide staining) was strongly induced by JQ1 treatment in U2OS and MNNG/HOS, but was only modestly increased in MG63 and unchanged in SaOS2 ( Fig. 2e ). Finally, apoptosis was evaluated in osteosarcoma cells by assessing the level of cleaved poly (ADP-ribose) polymerase after JQ1 treatment. Consistent with the results of the colony formation assays and cell cycle analysis, the same sensitivity profile was observed in the two cell lines with the lowest level of both BRD4 and MYC , namely, MNNG/HOS and U2OS were the most sensitive to apoptosis induction as revealed by the level of cleaved poly (ADP-ribose) polymerase, whereas two cell lines with a high level of BRD4 and MYC , namely, MG63 and SaOS2 were more resistant to the apoptotic effect of JQ1 ( Fig. 2f ). In addition, the induced apoptosis was confirmed in MNNG/HOS to be caspase-3 dependent ( Supplementary Fig. 4A ). These results confirmed our hypothesis that sensitivity of osteosarcoma tumours to BET bromodomains signalling inhibition is dependent on the expression level of BRD4 and MYC . We confirmed this hypothesis by the study of JQ1-resistant cell lines. We established MNNG/HOS-resistant cells by long-term exposure to increasing concentrations of JQ1. Once a significant difference in term of GI 50 could be observed, we performed quantitative reverse transcription (qRT)–PCR expression analysis for the BET bromodomains and MYC. As predicted by our hypothesis, we observed an overexpression of MYC and BRD4 in the resistant cell line, we also observed an overexpression of BRD2 but not BRD3 , suggesting a possible implication of several members of the BET bromodomain family in the mediation of JQ1 effects ( Supplementary Fig. 4B ). The sensitivity of murine osteosarcoma was also confirmed by the decrease in MYC expression, cell viability and colony formation in MOS-J, POS-1 and K7M2 cell lines ( Supplementary Fig. 4C,D ). 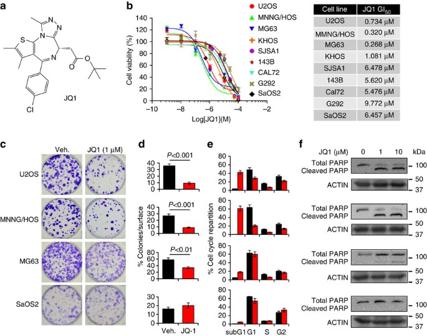Figure 2: JQ1 inhibits cell growth and induces apoptosis in human osteosarcoma cell lines. (a) Chemical structure of JQ1. (b) Human osteosarcoma cell lines (U2OS, MNNG/HOS, MG63, KHOS, SJSA-1, 143B, Cal72, G292 and SAOS2) were cultured for 72 h in the presence of JQ1 at the indicated concentration, and cell growth was determined by crystal violet assay and compared with control. GI50for JQ1 in tumour cell lines. (c) Osteosarcoma cells were treated with 1 μM JQ1 for 2 days, and then plated at clonal density for colony counts (d). (e) Osteosarcoma cells were treated with 1 μM JQ1 for 2 days, and the proportion of cells in subG1, G0–G1, S, G2–M was determined by propidium iodide staining. (f) Osteosarcoma cells were treated with 1 or 10 μM JQ1 for 2 days and apoptosis was evaluated by cleaved poly (ADP-ribose) polymerase (PARP) level by western blotting. All experiments were repeated at least twice. Error bars show s.e.m. forn=3 measurement from representative experiments. Figure 2: JQ1 inhibits cell growth and induces apoptosis in human osteosarcoma cell lines. ( a ) Chemical structure of JQ1. ( b ) Human osteosarcoma cell lines (U2OS, MNNG/HOS, MG63, KHOS, SJSA-1, 143B, Cal72, G292 and SAOS2) were cultured for 72 h in the presence of JQ1 at the indicated concentration, and cell growth was determined by crystal violet assay and compared with control. GI 50 for JQ1 in tumour cell lines. ( c ) Osteosarcoma cells were treated with 1 μM JQ1 for 2 days, and then plated at clonal density for colony counts ( d ). ( e ) Osteosarcoma cells were treated with 1 μM JQ1 for 2 days, and the proportion of cells in subG 1 , G 0 –G 1 , S, G 2 –M was determined by propidium iodide staining. ( f ) Osteosarcoma cells were treated with 1 or 10 μM JQ1 for 2 days and apoptosis was evaluated by cleaved poly (ADP-ribose) polymerase (PARP) level by western blotting. All experiments were repeated at least twice. Error bars show s.e.m. for n =3 measurement from representative experiments. Full size image MYC -dependent growth inhibitory effect of BET inhibition Since downregulation of MYC expression has been previously described as a consequence of BRD4 inhibition [19] , we accordingly examined the expression level of MYC after JQ1 treatment. In all the osteosarcoma cell lines tested, JQ1 treatment decreased MYC expression in a dose- and time-dependent manner ( Fig. 3a , Supplementary Fig. 5A,B ). We observed the same results in murine cell lines ( Supplementary Fig. 6 ). Indeed, after only 30 min of 0.5 μM JQ1, MYC expression was decreased by 30% in all cell lines studied, and 1 h of 0.1 μM JQ1 was sufficient to observe a significant effect ( Fig. 3a ). To confirm the functional impact of MYC transcriptional inhibition by JQ1, we assessed its effect on the expression of the MYC target gene mir-17–92 ( Fig. 3b ). After 24 h in the presence of 0.5 μM of JQ1, all seven microRNAs in the mir-17–92 cluster were significantly downregulated ( Fig. 3c ), Furthermore, p21, a direct target known to be repressed by the mir-17–92 cluster, was highly upregulated by 12-fold ( Fig. 3d and Supplementary Fig. 7A ). Interestingly, the rapid transcriptional effect of the BET inhibitor on MYC gene expression suggests the possibility that BET proteins may exert direct activation of the MYC locus. To determine whether BET proteins bind directly to the MYC locus, we performed chromatin immunoprecipitation (ChIP) studies by using an antibody targeting BRD4 in MNNG/HOS cells. We detected specific enrichment of BRD4 within the MYC promoter region at several locations including both upstream and downstream sites relative to the transcriptional start site ( Fig. 3e ). Furthermore, treatment of these cells with JQ1 induced the release of BRD4 from the promoter and binding sites ( Fig. 3e , bottom). The presence of DNAse hypersensitive sites and increased enrichment for histone 3 lysine 27 acetylation (H3K27ac) at the MYC promoter region indicates active transcription, perhaps associated with ‘super-enhancer region’ as recently described [28] , [29] . The specificity of the BRD4 antibody used in this study was assessed in a gene desert region that displayed no BRD4 enrichment. As mentioned for the resistance experiment, it looks like BRD2 (but not BRD3) might also be involved in the JQ1 effects on osteosarcoma. To validate our hypothesis, we performed the same ChIP at the MYC promoter region with a BRD2 antibody. While we observed an enrichment of BRD2 for the same regulatory areas as BRD4 on the MYC promoter region, no release of BRD2 was observed in the presence of JQ1. We even observed an opposite effect with a strong enrichment of BRD2 after JQ1 treatment. This effect is possibly due to the higher affinity of JQ1 for BRD4, interfering in the competition between BRD2 and BRD4 for the same binding sites. This effect did not lead to more MYC transcription, which is in agreement with the fact that neither BRD3 nor BRD2 were correlated with MYC expression in our patient cohort and BRD2 does not seem to be involved in JQ1 effects ( Supplementary Fig. 7B ). These findings demonstrate that BRD4 is present on the MYC promoter region and that JQ1 is able to deplete BRD4 from the promoter, thus inhibiting MYC transcription in an osteosarcoma cell line. Next, the growth-promoting activity of MYC was validated in our model using siRNA ( Fig. 3f ). To evaluate whether suppression of MYC mediates the growth inhibitory effect of BRD4 inhibition by JQ1, we performed a recovery assay by transfecting MYC or empty vector control into MNNG/HOS cells ( Fig. 3g ), followed by treatment with JQ1. Overexpression of MYC decreased significantly the anti-proliferative effect of JQ1 in osteosarcoma cells. Interestingly, it did not however inhibit fully the anti-proliferative effect of JQ1. 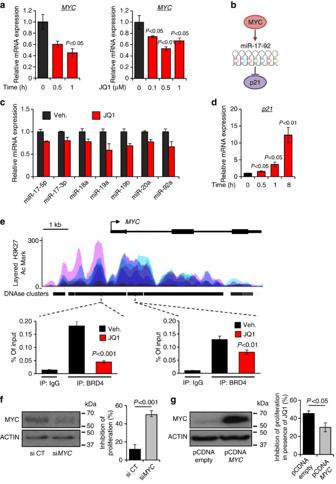Figure 3: Growth inhibition by JQ1 in osteosarcoma cells is dependent on MYC downregulation. (a) qRT–PCR for MYC RNA levels in JQ1-treated osteosarcoma cell line at (i) different time points (500 nM JQ1) and at (ii) different doses (1 h). analysis of variance (ANOVA), Bonferroni multiple comparisons statistical test has been used. (b) Schematic representation of the relationship betweenMYC,mir-17-92cluster andp21. (c) qRT–PCR for the mir-17-92 expression in JQ1-treated osteosarcoma cell (24 h, 0.5 μM JQ1). (d) qRT–PCR for p21 RNA levels in JQ1-treated osteosarcoma cell line (500 nM JQ1). ANOVA, Bonferroni multiple comparisons statistical test has been used. (e) ChIP with a BRD4 antibody at two sites within theMYCpromoter region in cells treated with 500 nM JQ1 for 4 h. Enrichment is shown as the percentage of total input DNA. The top track shows the levels of enrichment of the H3K27Ac histone mark across the genome as determined by a ChIP-seq assay on seven cell lines from ENCODE (f) Immunoblotting for MYC in siCT (control siRNA) or siMYC (MYCsiRNA) transfected MNNG/HOS cells and inhibition of cell proliferation in corresponding cells treated with JQ1 (500 nM, 72 h).t-test statistical analysis has been used. (g) Immunoblotting for MYC from empty pCDNA vector- orMYCoverexpression vector-transduced MNNG/HOS cells and inhibition of cell proliferation in corresponding cells treated with JQ1 (500 nM, 72 h),t-test statistical analysis has been used. Error bars show s.e.m. forn=3 measurement from representative experiments. Figure 3: Growth inhibition by JQ1 in osteosarcoma cells is dependent on MYC downregulation. ( a ) qRT–PCR for MYC RNA levels in JQ1-treated osteosarcoma cell line at (i) different time points (500 nM JQ1) and at (ii) different doses (1 h). analysis of variance (ANOVA), Bonferroni multiple comparisons statistical test has been used. ( b ) Schematic representation of the relationship between MYC , mir-17-92 cluster and p21 . ( c ) qRT–PCR for the mir-17-92 expression in JQ1-treated osteosarcoma cell (24 h, 0.5 μM JQ1). ( d ) qRT–PCR for p21 RNA levels in JQ1-treated osteosarcoma cell line (500 nM JQ1). ANOVA, Bonferroni multiple comparisons statistical test has been used. ( e ) ChIP with a BRD4 antibody at two sites within the MYC promoter region in cells treated with 500 nM JQ1 for 4 h. Enrichment is shown as the percentage of total input DNA. The top track shows the levels of enrichment of the H3K27Ac histone mark across the genome as determined by a ChIP-seq assay on seven cell lines from ENCODE ( f ) Immunoblotting for MYC in siCT (control siRNA) or si MYC (MYC siRNA) transfected MNNG/HOS cells and inhibition of cell proliferation in corresponding cells treated with JQ1 (500 nM, 72 h). t -test statistical analysis has been used. ( g ) Immunoblotting for MYC from empty pCDNA vector- or MYC overexpression vector-transduced MNNG/HOS cells and inhibition of cell proliferation in corresponding cells treated with JQ1 (500 nM, 72 h), t -test statistical analysis has been used. Error bars show s.e.m. for n =3 measurement from representative experiments. Full size image BET protein inhibition depletes BRD4 from the RUNX2 promoter As MYC downregulation did not account for all the anti-proliferative effect of JQ1, we then focused our attention on RUNX2 , a master transcription factor in osteosarcoma and OB. The expression level of RUNX2 was next evaluated in osteosarcoma patient samples compared with normal MSCs. We found that all the patient samples overexpressed RUNX2 ( Fig. 4a ). Moreover, we observed a strong correlation ( P <0.0001) between the expression levels of BRD4 and RUNX2 using the Pearson product-moment correlation coefficient ( R 2 ; Fig. 4b ). We validated this correlation in a lager cohort of 27 osteosarcoma patient biopsy samples obtained by Dr Yamada T from the National Cancer Center of Tokyo (GEO Series GSE14827) [27] . The expression array study confirmed the strong correlation between the expression levels of BRD4 and RUNX2 ( Supplementary Fig. 2 ). 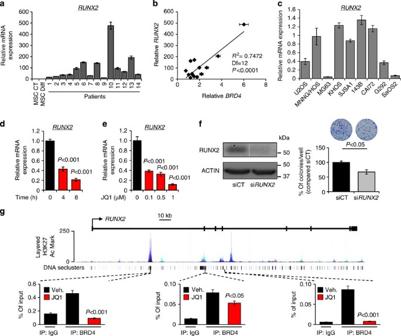Figure 4: The anti-tumoral activity of JQ1 involves the BRD4 depletion from the Runx2 promoter. (a) Expression ofRUNX2messenger RNA level was evaluated by qRT–PCR in human osteosarcoma biopsies compared with normal cells. (b) Correlation betweenBRD4andRUNX2expression in human osteosarcoma specimens, assessed by qRT–PCR and tested by the Pearson product-moment correlation test. (c) Expression ofRUNX2mRNA level in human osteosarcoma cell lines, assessed by qRT–PCR. (d,e) qRT–PCR forRUNX2RNA levels in JQ1-treated MNNG/HOS cell line at (d) different time points (500 nM JQ1) and at (e) different doses (8 h). Analysis of variance (ANOVA), Bonferroni multiple comparisons statistical test has been used. (f) Immunoblotting for RUNX2 from siCT (control siRNA) or siRUNX2(RUNX2 siRNA) transfected MNNG/HOS cells and then plated at clonal density for colony counts and inhibition of cell proliferation.t-test statistical analysis has been used. (g) ChIP with a BRD4 antibody at three sites around theRUNX2promoter region in cells treated with 500 nM JQ1 for 4 h. Enrichment is shown as the percentage of total input DNA. The top track shows the levels of enrichment of the H3K27Ac histone mark across the genome as determined by a ChIP-seq assay on seven cell lines from ENCODE. Error bars show s.e.m. forn=3 measurement from representative experiments. Figure 4: The anti-tumoral activity of JQ1 involves the BRD4 depletion from the Runx2 promoter. ( a ) Expression of RUNX2 messenger RNA level was evaluated by qRT–PCR in human osteosarcoma biopsies compared with normal cells. ( b ) Correlation between BRD4 and RUNX2 expression in human osteosarcoma specimens, assessed by qRT–PCR and tested by the Pearson product-moment correlation test. ( c ) Expression of RUNX2 mRNA level in human osteosarcoma cell lines, assessed by qRT–PCR. ( d , e ) qRT–PCR for RUNX2 RNA levels in JQ1-treated MNNG/HOS cell line at ( d ) different time points (500 nM JQ1) and at ( e ) different doses (8 h). Analysis of variance (ANOVA), Bonferroni multiple comparisons statistical test has been used. ( f ) Immunoblotting for RUNX2 from siCT (control siRNA) or si RUNX2 (RUNX2 siRNA) transfected MNNG/HOS cells and then plated at clonal density for colony counts and inhibition of cell proliferation. t -test statistical analysis has been used. ( g ) ChIP with a BRD4 antibody at three sites around the RUNX2 promoter region in cells treated with 500 nM JQ1 for 4 h. Enrichment is shown as the percentage of total input DNA. The top track shows the levels of enrichment of the H3K27Ac histone mark across the genome as determined by a ChIP-seq assay on seven cell lines from ENCODE. Error bars show s.e.m. for n =3 measurement from representative experiments. Full size image No correlation has been observed between RUNX2 and BRD2 or BRD3 using either our patient tumour samples or the larger Yamada’s lab cohort. Next, we evaluated the expression level of RUNX2 in different osteosarcoma cell lines and murine osteosarcoma cell lines. We observed an interesting variability, comparable to that observed within our patient cohort, which prompted us to study in greater detail the consequences of RUNX2 sensitivity to BET inhibition ( Fig. 4c and Supplementary Fig. 3 ). Interestingly, the two cell lines that express the highest level of RUNX2 (MNNG/HOS and U2OS) also express the lowest level of MYC , suggesting that different oncogenic processes may be driving these tumour cell lines ( Figs 1d and 4c ). We next investigated the expression level of RUNX2 after JQ1 treatment. In all the examined osteosarcoma cell lines, JQ1 treatment decreased RUNX2 expression in a time- and dose-dependent manner ( Fig. 4d,e and Supplementary Fig. 8A,B ). Similar to MYC , the growth-promoting activity of RUNX2 in osteosarcoma was validated in our cell model by siRNA knockdown and colony formation assay ( Fig. 4f ). Interestingly, we observed also the relatively fast transcriptional effects of BET inhibition on RUNX2 gene expression. This finding suggests that BET proteins might exert direct effects on the RUNX2 locus. To determine whether BET proteins bind directly to the RUNX2 locus, we performed ChIP studies by using an antibody against BRD4 in MNNG/HOS cells. While no enrichment of BRD4 within the RUNX2 promoter was detected, specific binding at the major H3K27 acetylated rich sites was observed ( Fig. 4g ). Treatment with JQ1 induced the release of BRD4 from these sites ( Fig. 4g ). The presence of DNAse clusters and the higher level of H3K27 acetylation in the identified binding sites indicate transcriptional activity and suggest the presence of a putative ‘super-enhancer region’ [28] , [29] . The specificity of the BRD4 antibody used in this study was also assessed in a gene desert region that displayed no BRD4 enrichment. For the same reasons as the MYC promoter, we performed a BRD2 ChIP for the RUNX2 locus. While we observed an enrichment of BRD2 for the same regulatory areas as BRD4 on the RUNX2 promoter region, no release of BRD2 could be observed in the presence of JQ1. We observed an opposite effect with a strong enrichment of BRD2 after JQ1 treatment ( Supplementary Fig. 8C ). To validate that the specificity of JQ1 effects on RUNX2 gene expression was mediated through the inhibition of BRD4-binding activity, we also assessed BRD4 enrichment at the IL7R locus following JQ1 treatment. IL7R is a recently described target of JQ1, BRD4 being removed from its promoter after treatment [22] . In our model, absolutely no BRD4 binding was detected at the IL7R promoter area with or without JQ1 treatment, confirming context-specific regulation of gene expression ( Supplementary Fig. 8D ). JQ1 delays osteosarcoma development and prolongs survival To investigate the in vivo therapeutic potential of BET inhibition in osteosarcoma, we used two models, a human xenograft model (using the MNNG/HOS cell line) and a syngeneic model (using the POS-1 cell line), both of which are known to recapitulate the features of the human disease. The POS-1 tumour cells were implanted in C3H mice while MNNG/HOS cells were injected in athymic mice at day 1 with 2 million cells in paratibial, and mice were then injected with JQ1 (50 mg kg −1 intraperitoneally (IP)) or vehicle twice a day for the indicated time. JQ1 treatment had a dramatic anti-tumoral effect, significantly reducing the average tumour volume in both mouse models. ( Fig. 5a,e ). Furthermore, the individual tumour volumes of treated mice compared with control group demonstrated a consistent effect of the treatment across the groups ( Fig. 5b,f ). Importantly, not a single treated mouse had a tumour progression over 1,000 mm 3 at day 20 and day 10 for the human and the mouse model, respectively, while all the untreated mice had tumours that exceeded that volume ( Fig. 5c,g ). In both models, the reduction in tumour volume obtained at the end of the experiment with JQ1 treatment was ~60%. The Kaplan–Meier analysis revealed that JQ1 treatment significantly prolonged survival of tumour-bearing mice. Incredibly, 100% of mice bearing MNNG/HOS tumour cells and 40% of mice bearing POS-1 cells were still alive with JQ1 treatment at the time when untreated mice were killed as their tumour volume reached institutional limits ( Fig. 5d,h ). Immunohistochemical staining for the proliferative marker Ki67 in tumour samples from mice showed that JQ1 treatment decreased cell proliferation as compared with the untreated cohort ( Fig. 5i ). Expression analysis for MYC and RUNX2 was also performed on these mice tumour samples. We observed a significant and reproducible repression of MYC and RUNX2 expression with JQ1 treatment, consistent with our in vitro results ( Fig. 5j ). Finally, as a functional validation for JQ1-mediated transcriptional repression of MYC in the mice tumour samples, we evaluated p21 expression ( Fig. 5j ). As expected, p21 expression was highly increased in the mice cohort treated with JQ1. Taken together, these data suggest that the potent in vivo anti-tumoral activity of JQ1 in osteosarcoma is probably mediated through its direct effects on the RUNX2 and MYC/p21 transcriptional network. 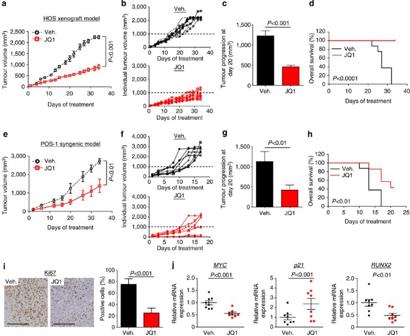Figure 5: JQ1 significantly delays tumour growth in MNNG/HOS xenograft and POS-1 syngeneic models and prolongs cancer-specific survival. Mice were IP injected with 50 mg kg−1JQ1 or vehicle (10% HP-β-CD) twice a day for the indicated time when tumour volume reached 100 mm3. The mean (a, human MNNG/HOS xenograft model ande, mouse POS-1 syngeneic model) or the individual (b,f) tumour volume of mice treated was compared with control group ±s.e.m. (respectively,n=8 orn=6). (c,g) The tumour progression was estimated as the relative tumour volumes (RTV) calculated from the formula: RTV=(V20−V1) whereV20is the mean tumour volume at day 20 andV1is the mean tumour volume at day 1 after starting treatment. (d,h) In Kaplan–Meier curves, cancer-specific survival were compared between mice treated with JQ1 and control. (i) Tumours were collected after 35 days (MNNG/HOS xenograft model) or 23 days (POS-1 model) and Ki67 was evaluated by immunohistochemical analysis (original magnification, × 200; scale bar, 200 μm). (j)MYC,p21andRUNX2were evaluated in tumour tissues, after RNA extraction, by qRT–PCR. Error bars show s.e.m. forn=3 measurement from representative experiments. Figure 5: JQ1 significantly delays tumour growth in MNNG/HOS xenograft and POS-1 syngeneic models and prolongs cancer-specific survival. Mice were IP injected with 50 mg kg −1 JQ1 or vehicle (10% HP-β-CD) twice a day for the indicated time when tumour volume reached 100 mm 3 . The mean ( a , human MNNG/HOS xenograft model and e , mouse POS-1 syngeneic model) or the individual ( b , f ) tumour volume of mice treated was compared with control group ±s.e.m. (respectively, n =8 or n =6). ( c , g ) The tumour progression was estimated as the relative tumour volumes (RTV) calculated from the formula: RTV=( V 20 − V 1 ) where V 20 is the mean tumour volume at day 20 and V 1 is the mean tumour volume at day 1 after starting treatment. ( d , h ) In Kaplan–Meier curves, cancer-specific survival were compared between mice treated with JQ1 and control. ( i ) Tumours were collected after 35 days (MNNG/HOS xenograft model) or 23 days (POS-1 model) and Ki67 was evaluated by immunohistochemical analysis (original magnification, × 200; scale bar, 200 μm). ( j ) MYC , p21 and RUNX2 were evaluated in tumour tissues, after RNA extraction, by qRT–PCR. Error bars show s.e.m. for n =3 measurement from representative experiments. Full size image JQ1 prevents osteosarcoma tumour-associated bone deficiencies We next examined the effects of JQ1 on the bone microarchitecture of tumour-bearing tibia from mice injected with MNNG/HOS cells using microcomputed tomography (microCT; Fig. 6a ) followed by three-dimensional reconstruction ( Fig. 6b ). Surprisingly, JQ1 treatment preserved the bone microarchitecture as there was a marked reduction in tumour-associated osteolysis, a common feature of tumour-bearing bone ( Fig. 6a,b ). An extensive analysis of multiple bone morphometric parameters revealed a strong and significant amelioration of tumour-associated bone quality in the JQ1-treated group. Indeed, JQ1 treatment prevented destruction of the trabecular bone and improved the trabecular bone volume (BV/TV) from 3 to 13% ( Fig. 6c ), the trabecular number (per mm) from 0.5 to 1.6 ( Fig. 6d ), the trabecular thickness (mm) from 0.06 to 0.08 ( Fig. 6e ) and decreased the trabecular separation (mm) from 0.57 to 0.41 ( Fig. 6f ). One characteristic of osteosarcoma tumours is the formation of ectopic bone. Our analysis using microCT showed a strong decrease of this ectopic bone formation in the presence of JQ1 on the tumour-bearing tibia, with an average of only 0.13 mm 3 against 1.73 mm 3 in the vehicle group ( Fig. 6g,h ). Histological analysis of the tumour-bearing bone with tartrate-resistant acid phosphatase (TRAP) and Osterix staining revealed that JQ1 treatment strikingly decreased the number of OCs as well as the number of OBs ( Fig. 6i,j ). The same bone morphometric analysis was also conducted on tumour-bearing tibia from the syngeneic mouse model and similar results in bone quality improvement were observed in the JQ1-treated cohort ( Supplementary Fig. 9 ). 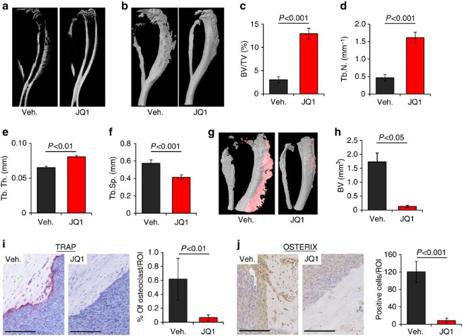Figure 6: BRD4 inhibition prevents MNNG/HOS tumour bone loss. Representative microCT (a) and three-dimensional model (b) images of the tumour-bearing tibia, takenex vivo, from MNNG/HOS-bearing mice treated with JQ1 (50 mg kg−1) or vehicle (Veh.). (c–f) MicroCT analysis of the BV/TV (%) (c), trabecular number (Tb.N (per mm)) (d), trabecular thickness (Tb.Th (mm)) (f) and trabecular separation (Tb.Sp (mm)) of the tibia of tumour-bearing mice treated JQ1 or vehicle. (g) Representative images of the ectopic bone (red) of tumour-bearing tibia, takenex vivo, from MNNG/HOS-bearing mice treated with JQ1 (50 mg kg−1) or vehicle (Veh.). (h) MicroCT analysis of the ectopic BV (mm3). TRAP (i) and Osterix (j) were evaluated by immunohistochemical analysis (original magnification, × 200; scale bar, 200 μm). Specimens were scored and estimated in % of positive cells ±s.d. for OSTERIX, and the surface occupied by OC was determined by ImageJ in the delimited region of interest (ROI). Error bars show s.e.m. forn=3 measurement from representative experiments. Figure 6: BRD4 inhibition prevents MNNG/HOS tumour bone loss. Representative microCT ( a ) and three-dimensional model ( b ) images of the tumour-bearing tibia, taken ex vivo , from MNNG/HOS-bearing mice treated with JQ1 (50 mg kg −1 ) or vehicle (Veh.). ( c – f ) MicroCT analysis of the BV/TV (%) ( c ), trabecular number (Tb.N (per mm)) ( d ), trabecular thickness (Tb.Th (mm)) ( f ) and trabecular separation (Tb.Sp (mm)) of the tibia of tumour-bearing mice treated JQ1 or vehicle. ( g ) Representative images of the ectopic bone (red) of tumour-bearing tibia, taken ex vivo , from MNNG/HOS-bearing mice treated with JQ1 (50 mg kg −1 ) or vehicle (Veh.). ( h ) MicroCT analysis of the ectopic BV (mm 3 ). TRAP ( i ) and Osterix ( j ) were evaluated by immunohistochemical analysis (original magnification, × 200; scale bar, 200 μm). Specimens were scored and estimated in % of positive cells ±s.d. for OSTERIX, and the surface occupied by OC was determined by ImageJ in the delimited region of interest (ROI). Error bars show s.e.m. for n =3 measurement from representative experiments. Full size image BET inhibition interferes with the OC and OB differentiation Given the surprisingly strong effects of BET bromodomain proteins inhibition on the bone-microarchitecture, tumour-associated osteolysis and OC as well as OB number in the tumour bearing bone, we further evaluated the possible effect of JQ1 on OC and OB differentiation. First, purified human CD14 + monocytes were cultured in the presence of human macrophage colony stimulating factor and hRANKL to induce osteoclastic differentiation as well as in the presence or absence of JQ1. Subsequently, TRAP coloration was performed and the number of multinucleated cells was assessed ( Fig. 7a ). BET bromodomain protein inhibition by JQ1 treatment indeed blocked OC differentiation by more than 80% ( Fig. 7b ). This block in OC differentiation by JQ1 appears to be independent of its effect on cell proliferation and survival as it had virtually no effect on the cell viability of OC precursors. ( Supplementary Fig. 10 ). To begin to identify the underlying mechanism of JQ1-mediated inhibition of OC differentiation, we first tested the activity of NFkB using a luciferase-based reporter construct containing its consensus binding site. Cells expressing RANK were transfected with the NFkB promoter construct and were then treated with RANKL in the presence or absence of JQ1. Our results show that treatment with JQ1 suppressed by more than 50% RANKL-stimulated NFkB transcriptional activity ( Fig. 7c ). We then confirmed the suppressive effect of JQ1 on NFkB activity by examining the expression of NFkB target genes that are known to be associated with the differentiation process of OC. JQ1 not only decreased the expression of NFkB target genes NFATC1 and MMP9 but also completely abrogated the expression of calcitonin receptor, a marker of OC differentiation in OC precursors cultured with RANKL ( Fig. 7d–f ). Consistent with these findings, ChIP analysis confirmed the presence of BRD4 at several NFkB-binding sites on the NFATC1 and MMP9 promoters. Moreover, we demonstrated enrichment of BRD4 only when NFkB was activated by RANKL and that JQ1 was able to deplete BRD4 from these promoters in RANKL-stimulated OC precursors. As suggested above, BRD2 might be implicated in the JQ1 effects; this hypothesis is even more relevant in the case of NFkB-dependent promoter like NFATC1 and MMP9 because significant published evidence shows that BRD2 has a non-redundant, BRD4-independent role in proliferation and inflammation regulating NFkB target genes, for instance IL-6 and tumour necrosis factor-α transcription [30] . We performed a BRD2 ChIP looking at several NFkB-binding sites on the NFATC1 and MMP9 promoters. While we demonstrated a RANKL-dependent enrichment of BRD2 on the NFkB-binding sites, no significant depletion of BRD2 in presence of JQ1 could be observed ( Supplementary Fig. 11 ). Altogether, these data indicate that JQ1 likely inhibits pro-osteoclastic differentiation through interference with BRD4-dependent RANKL activation of NFATC1 and MMP9 transcription ( Fig. 7g and Supplementary Fig. 12 ). Next, we interrogated the effect of JQ1 on OB differentiation using human MSCs cultured in OB differentiation medium as well as in the presence or absence of JQ1. After 21 days, we assessed OB differentiation by evaluating the extent of mineralization staining with Alizarin red. JQ1 treatment resulted in a marked decrease by 60% in mineralization staining, indicating that BRD4 inhibition blocks OB differentiation ( Fig. 7h ). This inhibition of OB differentiation by JQ1 is completely independent of its effect on cell proliferation/survival as revealed by cell viability assays ( Supplementary Fig. 13A ). Then, we examined the expression of RUNX2 , which plays a critical role in OB differentiation, in addition to the expression of ALP (alkaline phosphatase), a marker of the osteoblastogenesis. JQ1 treatment leads to significant reduction in RUNX2 and ALP gene expression, emphasizing the inhibitory effect of JQ1 at the transcriptional level ( Fig. 7i,j ). This finding is consistent with our previous results showing that BRD4 was detected at the RUNX2 DNA locus and that JQ1 was able to deplete BRD4 from those sites ( Fig. 4g ). Taken together, these data indicate that BRD4 inhibition with JQ1 blocks both osteoclastogenesis and osteoblastogenesis in vitro and in vivo . Finally and equally importantly, we found that microCT analysis of normal bone following JQ1 treatment showed no significant adverse effects on bone morphometric parameters ( Supplementary Fig. 13B–F ). 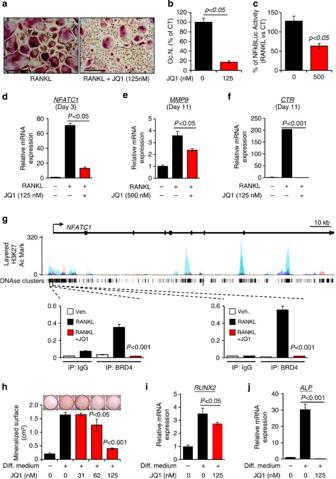Figure 7: BRD4 inhibition inhibits bone cells differentiation. (a,b) Purified human CD14+monocytes were cultured for 13 days in the presence of M-CSF, RANKL and JQ1. TRAP colouration was performed at the end of the culture period (a) and multinucleated TRAP-positive cells were counted under a light microscope (scale bar, 100 μm) (b),t-test statistical analysis has been used. (c) Activity of the transcription factor NFkB as assessed with a luciferase report assay. HEK293-RANK were transfected with NFkB-Luc vector and then treated with and JQ1 (500 nM) for 24 h. Results show relative luciferase units (RLU, in %) normalized to the condition without RANKL. (d–f) qRT–PCR forNFATC1(d),MMP9(e) andCTR(calcitonin receptor) (f) RNA levels in human CD14+monocytes cultured in the presence of M-CSF, RANKL and 125 nM JQ1 after 3 days (d) or 11 days (e,f). Analysis of variance (ANOVA), Bonferroni multiple comparisons statistical test has been used. Results are expressed as fold increase compared with the condition without RANKL and JQ1. (g) ChIP with a BRD4 antibody at two sites around theNFATC1promoter region in cells treated with 500 nM JQ1 for 4 h and RANKL (100 ng ml−1) for 1 h. Enrichment is shown as the percentage of total input DNA. The top track shows the levels of enrichment of the H3K27Ac histone mark across the genome as determined by a ChIP-seq assay on seven cell lines from ENCODE. (h–j) Human MSCs were cultured in OB differentiation medium (Diff. medium) and treated with JQ1. After 21 days, mineralization was quantified after staining with alizarin red-S (h). Expression ofRUNX2(i) andALP(alkaline phosphatase) (j) RNA levels were assessed by qRT–PCR. Results are expressed as fold increase compared with the control condition without differentiation medium. ANOVA, Bonferroni multiple comparisons statistical test has been used. Error bars show s.e.m. forn=3 measurement from representative experiments. Figure 7: BRD4 inhibition inhibits bone cells differentiation. ( a , b ) Purified human CD14 + monocytes were cultured for 13 days in the presence of M-CSF, RANKL and JQ1. TRAP colouration was performed at the end of the culture period ( a ) and multinucleated TRAP-positive cells were counted under a light microscope (scale bar, 100 μm) ( b ), t -test statistical analysis has been used. ( c ) Activity of the transcription factor NFkB as assessed with a luciferase report assay. HEK293-RANK were transfected with NFkB-Luc vector and then treated with and JQ1 (500 nM) for 24 h. Results show relative luciferase units (RLU, in %) normalized to the condition without RANKL. ( d – f ) qRT–PCR for NFATC1 ( d ), MMP9 ( e ) and CTR (calcitonin receptor) ( f ) RNA levels in human CD14 + monocytes cultured in the presence of M-CSF, RANKL and 125 nM JQ1 after 3 days ( d ) or 11 days ( e , f ). Analysis of variance (ANOVA), Bonferroni multiple comparisons statistical test has been used. Results are expressed as fold increase compared with the condition without RANKL and JQ1. ( g ) ChIP with a BRD4 antibody at two sites around the NFATC1 promoter region in cells treated with 500 nM JQ1 for 4 h and RANKL (100 ng ml −1 ) for 1 h. Enrichment is shown as the percentage of total input DNA. The top track shows the levels of enrichment of the H3K27Ac histone mark across the genome as determined by a ChIP-seq assay on seven cell lines from ENCODE. ( h – j ) Human MSCs were cultured in OB differentiation medium (Diff. medium) and treated with JQ1. After 21 days, mineralization was quantified after staining with alizarin red-S ( h ). Expression of RUNX2 ( i ) and ALP (alkaline phosphatase) ( j ) RNA levels were assessed by qRT–PCR. Results are expressed as fold increase compared with the control condition without differentiation medium. ANOVA, Bonferroni multiple comparisons statistical test has been used. Error bars show s.e.m. for n =3 measurement from representative experiments. Full size image The vicious cycle established between bone-associated tumours and bone resorption is the fundamental pathophysiologic feature of both primary bone tumours and bone metastasis [1] , [5] . While therapeutic interventions have been developed to disrupt the vicious cycle of bone cancer, none to our knowledge targets all three partners of this cycle, the bone-associated tumours, OB and OCs. For example, clinical treatment with the bisphosphonate zoledronic acid induces apoptosis in OC and in some reports cell death in the tumour cells [31] , while treatment with the anti-RANKL monoclonal antibody denosumab inhibits OCs [32] . In this study, we uncover an essential role of BET bromodomain signalling in the vicious cycle as inhibition of BET bromodomain signalling not only potently suppresses the proliferation of bone-associated tumour cells but the differentiation of both OB and OC as well. Thus, our work is the first to support BET bromodomain inhibition as a therapeutic strategy to simultaneously target all three partners of the vicious cycle, which suggest that this approach may yield better therapeutic efficacy than standard treatments for primary and secondary bone cancer. Since the recent discovery that BET proteins act as mediators in the epigenetic recognition of acetylated lysines to regulate chromatin accessibility, it has become an increasingly attractive therapeutic target in several types of cancer [19] , [20] , [21] , [22] , [26] . Here we report for the first time data to support bromodomain inhibition as a therapeutic strategy for bone-associated tumours. Using the unique BET protein inhibitor JQ1, we demonstrate potent activity against a range of human and mouse osteosarcoma cell lines as well as in osteosarcoma preclinical models. We observe a strong reduction in cell viability of osteosarcoma cells with BET bromodomain inhibition irrespective of whether the oncogenic ‘driver’ was MYC or RUNX2 . Furthermore, it should be noted that the reduction of MYC gene expression does not fully account for the anti-proliferative effect of BET inhibition, as exogenous expression of MYC could not completely abolish the growth inhibitory effect of JQ1. This observation led us to the finding that BET inhibition also resulted in the downregulation of RUNX2 gene expression in osteosarcoma cells. This finding is of clinical relevance, given the emerging role of RUNX2 as a potential oncogene in osteosarcoma [12] , [13] , [14] , [15] , [16] . In addition, we found that RUNX2 gene expression, as well as that of MYC and BRD4 , was higher relative to MSCs in the majority of our human osteosarcoma patient samples suggesting an addiction or at least a dependence to those oncogenes. This makes most osteosarcoma patients likely to be sensitive to this BRD4- , MYC- and RUNX2 -dependent therapeutic strategy. In our model, BRD4 actively binds to both MYC and RUNX2 gene loci, specifically at the sites of highly acetylated H3K27. In support of this, we observe that transcriptional silencing of MYC and RUNX2 following JQ1 treatment is associated with the release of BRD4 proteins from their corresponding loci, indicating that BET proteins directly regulate the expression of MYC and RUNX2 genes. Moreover, BRD4 is released from the acetylated histones of the MYC and RUNX2 gene loci in response to JQ1 treatment, consequently leading to their reduced gene expression. While we observed striking anti-tumoral activity against primary bone tumours in vivo with BET inhibition, resulting in prolonging overall survival as well as improving tumour-associated bone structural parameters, JQ1 had virtually no adverse effects on normal bone architecture. Although BRD4 is expressed in almost all tissues, no overt toxicity was detected with high doses of JQ1. Indeed, repeated treatments with JQ1 did not result in weight loss or other negative effects during the course of the experiment. This highlights the importance of understanding how the inhibition of a ubiquitous regulator like BRD4 can have such a gene-specific effect on transcription. Interestingly, recent studies have identified an asymmetric distribution of BRD4 at enhancer regions across the epigenome, the so-called super-enhancers have a high: density of transcription factors, ability to activate transcription, levels of H3K27 acetylation and sensitivity to perturbation by BET bromodomain inhibition [28] , [29] . These super-enhancers are described to be associated with key cell type-specific genes known to play prominent roles in the biology of normal cells, and with oncogenic drivers in tumour cells. Furthermore, JQ1 treatment of multiple myeloma tumour cells caused the preferential loss of BRD4 at super-enhancers and preferential loss of transcription at super-enhancer-associated genes including the MYC oncogene. The mechanistic explanation of this phenomenon is based on the behaviour of regular enhancer regions, where cooperative and synergistic binding of multiple transcription factors can occur. The more cooperatively interacting factors there are bound on enhancers, the more sensitive these enhancers are to small changes in transcription factor concentration [33] , [34] , [35] . Consequently, super-enhancer regions are extremely sensitive to reduced level of BRD4, which could possibly explain the gene-selective effects of JQ1. It is very likely that the new target of JQ1 identified in our study, namely, RUNX2 , fit the definition of a super-enhancer. RUNX2 is not only a key cell type gene for OB but also a potential oncogenic driver for osteosarcoma. Moreover, we observe on ENCODE a high level of H3K27 acetylation mark along with a very high density of transcription factor-binding sites at the BRD4 binding sites of the RUNX2 locus. An unexpected finding was the effect of BET inhibition on OC differentiation. We observed that JQ1 inhibited NFkB activity without altering its transcription. NFkB is the key upstream regulator of osteoclastogenesis, directly activated by RANK after RANKL binding, and one of its primary transcriptional targets is the transcription factor NFATC1. Under basal condition, we did not detect binding of BRD4 to the NFATC1 promoter irrespective of the level of H3K27 acetylation, emphasizing the possible absence of BRD4 at some gene promoters. However, on RANKL activation, we observed strong binding of BRD4 onto the NFATC1 promoter at the precise NFkB consensus sites previously reported [36] . Our interpretation of these results is that BRD4 functions as a co-activator of NFkB via specific binding to its acetylated RelA subunit. Indeed, BRD4 has been identified as a co-activator of NFkB through its binding to the acetylated lysine-310 of RelA [37] , [38] . In agreement with this, we also found that JQ1 abrogated BRD4 binding to NFkB consensus sites on the NFATC1 promoter as well as inhibited osteoclastogenesis. Similar results were also found with MMP9, an OC functional protein. Taken together, our results indicate that BRD4 is an essential regulator of osteoclastogenesis and highlights the requirement for BRD4 in regulating MYC and RUNX2 through one specific mechanism, and NFATC1 through a completely different mechanism. In conclusion, pharmacological inhibition of BET bromodomain proteins appears to be a promising and relevant strategy for the treatment of bone-associated tumours as it interferes with the vicious cycle between bone tumour development and bone remodelling. Importantly, JQ1 becomes the first described compound to inhibit simultaneously bone tumour growth as well as both OB and OC differentiation. The ability of the BET inhibitor JQ1 to target all three major components of the vicious cycle makes it potentially less sensitive to develop treatment resistance, an aspect that we will further investigate ( Fig. 8 ). This triple inhibitory effect associated with low toxicity in vivo makes JQ1 a promising therapeutic agent for the treatment of both primary bone tumours and bone metastasis. 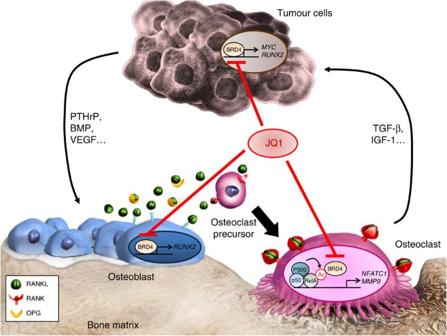Figure 8: BET bromodomain inhibition as a new therapeutic strategy to block the vicious cycle in bone tumours. The vicious cycle described in primary bone tumours and bone metastases consists of release of osteolytic mediators by tumour cells and OBs, thus inducing bone degradation and then releasing growth factors from degraded bone, enhancing tumour cell growth and further release of osteolytic mediators. In the present study, we describe for the first time the therapeutic interest of BET bromodomain inhibitor, JQ1, in the treatment of osteosarcoma not only by the prevention of osteosarcoma-induced osteolysis by blocking both OC and OB differentiation, but also by the inhibition of associated tumour development, leading to increased survival rate. Figure 8: BET bromodomain inhibition as a new therapeutic strategy to block the vicious cycle in bone tumours. The vicious cycle described in primary bone tumours and bone metastases consists of release of osteolytic mediators by tumour cells and OBs, thus inducing bone degradation and then releasing growth factors from degraded bone, enhancing tumour cell growth and further release of osteolytic mediators. In the present study, we describe for the first time the therapeutic interest of BET bromodomain inhibitor, JQ1, in the treatment of osteosarcoma not only by the prevention of osteosarcoma-induced osteolysis by blocking both OC and OB differentiation, but also by the inhibition of associated tumour development, leading to increased survival rate. Full size image Tumour cell line and patient tumour material The human osteosarcoma cell lines MG63 (young male osteosarcoma), SaOS2 (young female osteosarcoma), U2OS (young female osteosarcoma from tibia origin), MNNG/HOS (young female high-grade osteosarcoma from femur origin transformed in vitro by N -methyl- N ′-nitro- N -nitrosoguanidine treatment), KHOS (this cell line was derived from HOS by transformation using Kirsten murine sarcoma virus (Ki-MSV), SJSA-1 (was established in 1982 from the primary tumour of a patient diagnosed with primitive multipotential sarcoma of the femur, there is amplification of the gene that encodes the p53-associated protein, MDM2, SJSA-1 cells also exhibit a 15-fold amplification of the gli proto-oncogene), 143B (13 years old Caucasian female, thymidine kinase negative) G-292 (young female osteosarcoma), CAL 72 (osteosarcoma of the knee of a 10-year-old boy) and the murine osteosarcoma cell lines POS-1 and MOS-J were purchased from the American Type Culture Collection and maintained in DMEM (Invitrogen-Life Technologies Inc.) supplemented with 10% fetal bovine serum and 2 mmol l −1 L -glutamine. All cell lines were cultured in a humidified 5% CO 2 /air atmosphere at 37 °C. All cell lines were passaged for less than 3 months. Patient tumour biopsy specimens were collected at Nantes University Hospital (Nantes, France). Samples were obtained following patient informed consent, and after ethical approval by the Nantes University Hospital Ethics Committee. Therapeutic agents Brd4 inhibitor, JQ1, was kindly provided by James Bradner (Dana-Farber Cancer Institute). This synthetic compound targets selectively the acetyl-lysine-binding pocket of the BET bromodomain proteins. For in vitro studies, JQ1 was dissolved in dimethyl sulphoxide at 10 mM stock solutions and stored at −20 °C. For the in vivo studies, JQ1 was dissolved in dimethyl sulphoxide at 50 mg ml −1 and then diluted in 10% hydroxypropyl beta cyclodextrin (HP-β-CD, Sigma-Aldrich) to get the final dose, 50 mg kg −1 and stored at 4 °C. The 10% HP-β-CD is prepared in sterile water, which was filtered with 0.22 μ filter. MYC expression vector and siRNA Coding sequence for human MYC was cloned into the expression vector pCDNA3 (Life Technologies). Transfection was performed using Jet-PEI, according to the manufacturer’s recommendations (Polyplus-Transfection, Illkirch, France). For siRNA, cells were transfected with Interferin (Polyplus-Transfection) and annealed siRNA (20 nM); (si MYC (s9129 from Ambion, Applied Biosystems, Courtaboeuf, France) and si RUNX2 (HSS101403 from Life Tecnologies)), according to the manufacturer’s recommendations. Cell proliferation and apoptosis assays Osteosarcoma cell lines were plated in DMEM with 5% FBS and treated with JQ1 at indicated concentration, and time and cell growth was measured using the crystal violet assay as described previously. Detection and quantitation of dead cells were done by flow cytometry (described below) and western blotting analysis. Each assay was repeated in triplicate. Cell cycle analysis Osteosarcoma cell lines were incubated in the absence or the presence of 1 μM JQ1 for 72 h, trypsinized, washed twice and incubated in PBS containing 0.12% Triton X-100, 0.12 mM EDTA and 100 μg ml −1 ribonuclease A; 50 μg ml −1 propidium iodide was then added to each sample for 20 min at 4 °C. Cell cycle distribution was analysed by flow cytometry (Cytomics FC500; Beckman Coulter, Roissy, France) based on 2N and 4N DNA content. Each assay was done in triplicate. Western blotting analysis Samples containing equal amounts of protein (depending on the antibody, 5–50 μg) from lysates of cultured osteosarcoma cell lines underwent electrophoresis on SDS–PAGE and were transferred to polyvinylidene difluoride membranes. The membranes were blocked in 3% BSA–PBS-0.1% Tween at room temperature for 1 h and blots were probed overnight at 4 °C with primary antibodies (MYC and RUNX2, 1:1,000; Cell Signaling Technologies, Beverly, CA) or actin (1:20,000; Sigma-Aldrich) to detect proteins of interests. After incubation, the membranes were washed three times with washing buffer (PBS containing 0.1% Tween) for 5 min. Membranes were then incubated for 1 h with 1:10,000 diluted secondary antibodies (Santa Cruz Biotechnologies, Santa Cruz, CA) at room temperature. Specific proteins were detected using G-Box (Syngene, Cambridge, UK) after washing. Uncropped scans of the most important western blots are provided as Supplementary Figs 14–16 . Quantitative reverse transcription–PCR Total RNA was extracted from cultured cells, human biopsies or xenografts using TRIreagent (Invitrogen-Life Technologies Inc.). Total RNA was reversed transcribed using the ThermoScript RT–PCR System (Life Technologies). Real-time monitoring of PCR amplification of complementary DNA was performed using DNA primers (primers sequences are available in Supplementary Table 1 ) on CFX96 real-time PCR detector system (Bio-Rad, Marnes la Coquette, France) with SYBR PCR Master Mix buffer (Bio-Rad). Target gene expression was normalized to glyceraldehyde 3-phosphate dehydrogenase levels in respective samples as an internal standard, and the comparative cycle threshold method was used to calculated relative quantification of target messenger RNAs. Each assay was performed in triplicate. qRT–PCR microRNA A specific RT was performed for each miR from 100 ng of total RNA, using a specific stem-loop RT primer (50 nM) and the MultiScribe Reverse transcriptase (Applied Biosystems). The RT conditions were as follows: 30 min at 16 °C followed by 30 s at 20 °C, 30 s at 42 °C, 1 s at 50 °C for 60 cycles, and finally 5 min at 85 °C. Mature microRNAs’ expression levels were measured by real-time qRT–PCR using the SYBR PCR Master Mix buffer (Bio-Rad) and an CFX96 real-time PCR detector system (Bio-Rad). The expression of each gene was normalized to the small nuclear U6B RNA or 5S ribosomal RNA as a reference. All experiments were performed in triplicate. Primers sequences are available in Supplementary Table 2 . Quantitative ChIP assay A ChIP assay was performed by the Magnify ChIP system (Invitrogen-Life Technologies Inc.) using 5 μg of BRD4 antibody (Bethyl Lab) or control rabbit IgG (R&D Systems). Real-time PCR (Bio-Rad) was performed on fragmented DNA using specific primers for the MYC , RUNX2 , NFATC1 , MMP9 and IL7R loci. Primers were designed to amplify sites within each gene locus based on the H3K27 acetylation level, and a negative control region was designed outside the promoter region (primers sequences are available in Supplementary Table 3 ). The levels of enrichment of the H3K27Ac histone mark across the genome has been determined by a ChIP-seq assay on seven cell lines from ENCODE web resourses. Luciferase assay The cell line HEK293 overexpressing RANK was obtained by transducing cells with lentivirus containing the coding sequence of RANK and were then selected with antibiotic selection. HEK293-RANK cells were seeded in 24-well plates and were transfected with the indicated firefly luciferase constructs (pNF-kB-Luc reporter, BD Biosciences, Clonetech) together with an SV40-renilla control vector. Lysates were prepared at 40 h, and luciferase activity was measured using the Dual Luciferase Reporter Assay system (Promega) and a luminometer (MicroLumat Plus; EG&G Berthold). OC differentiation OCs were generated from human CD14+ monocytes. Purified CD14+ cells were cultured in α-MEM with 10% FCS and 25 ng0060ml −1 human macrophage colony stimulating factor (R&D Systems). After 4 days of culture, 100 ng ml −1 hRANKL and 125 nM JQ1 were added. Multinucleated cells formed with three nuclei and more were counted after TRAP staining (Sigma, France) [39] . OB differentiation Before passage 5, MSCs were seeded at 10 4 cells per cm 2 in 96-well plates in DMEM supplemented with vitamin D3 (10 −8 M; Hoffmann-La Roche, Basel, Switzerland), dexamethasone (10 −8 M; Sigma) and with or without JQ1 as indicated (this represented day 0 for MSC osteogenic differentiation). Three days later, freshly prepared ascorbic acid (50 μg ml −1 ; Sigma) and β-glycerophosphate (10 mM; Sigma) was added to allow mineralization, this medium being changed every 2–3 days. Alizarin red-S staining was used to detect the mineralized nodules formed in vitro as described previously [40] . In brief, between day 19 and 21, cells were fixed in ice-cold 70% ethanol for 1 h and incubated with alizarin red-S (40 mM, pH 7.4; Sigma) for 10 min at room temperature. After extensive washing, images were captured using a stereo microscope (Stemi 2000-C; Zeiss, Oberkochen, Germany, http://www.zeiss.com ), and mineralized surfaces were quantified using the Qwin software (Leica, Nussloch, Germany, http://www.leica-microsystems.com ). Animal treatment All procedures involving mice (their housing in the Experimental Therapeutic Unit at the Faculty of Medicine of Nantes (France) and care, the method by which they were anaesthetized and killed, and all experimental protocols) were conducted in accordance with the institutional guidelines of the French Ethical Committee (CEEA.PdL.06). Mice were anaesthetized by inhalation of a combination of isoflurane/air (1.5%, 1 l min −1 ) and buprenorphine (0.05 mg kg −1 ; Temgésic, Schering-Plough). Tumour volume was measured three times weekly and tumour volume was calculated by using the formula: length × width × depth × 0.5432. Data points were expressed as average tumour volume ±s.e.m. HOS osteolytic xenograft model was induced by an intramuscular injection of 2 × 10 6 human HOS cells next to the tibia of 5-week-old female athymic nude mice (Harlan Sprague–Dawley Inc.), leading to a rapidly growing tumour in soft tissue with secondary contiguous bone invasion. Once palpable tumours, mice were randomly assigned to vehicle or JQ1. When tumours reached 100 mm 3 , JQ1 (50 mg kg −1 ; formulation in 10% HP-β-CD in sterile water) is IP injected twice a day, every day. Each experimental group consisted of eight mice. To establish syngenic POS-1 tumour model, 5-week-old male C3H/He mice were anaesthetized before subcutaneous inoculation of POS-1 cell suspension (containing 2 × 10 6 cells) in the hind footpad of the mice. Under these conditions, mice develop a primary tumour at the site of injection in 3 weeks that can be transplanted to mice of the same strain as a small fragment (2 × 2 × 2 mm 3 ) in close contact with the tibia. For this purpose, the periostum of the diaphysis was opened and resected along a length of 5 mm, and the underlying bone was intact. The osteosarcoma fragment was placed contiguous to the exposed bone surface without the periostum, and the cutaneous and muscular wounds were sutured. Tumours appeared at the graft site ~8 days later associated with the development of pulmonary metastases in a 3-week period. The tumours that develop in contact to the femora lead to osteolytic lesions that reproduce the osteolytic form of human osteosarcoma [41] . When tumours reached 100 mm 3 , mice were randomly selected for treatment with vehicule or JQ1 (50 mg kg −1 ). JQ1 was injected I.P twice a day, every day. Each experimental group consisted of six mice. When tumour volume reached ⩾ 10% of body weight, mice were killed and tumours harvested for evaluation of protein expression by western blotting analyses and immunohistochemistry. MicroCT analysis MicroCT analysis has been previously described [42] . In brief, tibias were scanned using high-resolution microcomputed tomography (Skyscan 1076, Kontich, Belgium) at 50 kV and 200 μA using a 0.5-mm aluminium filter and a detection pixel size of 9 μm. Images were captured every 0.6° through 180° rotation, and analysed using Skyscan software. Trabecular structures positioned 0.2 mm below the growth plate were quantified over a length of 1 mm. BV/TV, trabecular thickness, trabecular separation and Tb.N. were determined. The BV of ectopic bone was quantified over the total length of tibia bearing tumour. Bone histomorphometric analysis and immunohistochemistry Tibias were decalcified with 4.13% EDTA and 0.2% paraformaldehyde in PBS for 96 h using the KOS microwave histostation (Milestone, Kalamazoo, MI, http://www.milestonemed.com ) before embedding in paraffin. Sections (3 μm thick, Leica Microsystems) were analysed by TRAP staining as described previously [43] , [44] . Immunostaining for Osterix was performed as described [43] with a rabbit anti-osterix antibody (1/25; Abcam, Cambridge, MA, http://www.abcam.com ). Quantification of relative OC surface (TRAP+ cells) and OB number (osterix+cells) in the metaphyseal spongiosa was evaluated by Qwin (Leica) and ImageJ (NIH, Bethesda, MD) softwares. Immunostaining for Ki67 was conducted using a primary antibody mouse anti-human Ki67 (1:100; Dako) on tumour section. All analyses were assessed by light microscopy using a DMRXA microscope (Leica). All comparisons of staining intensities were made at × 200 magnifications. Statistical analysis For each experimental data point, the s.e.m. from replicate experiments was calculated as noted in the legends and is shown as error bars. All error bars show s.e.m. for at least triplicate measurement from representative experiments. The mean±s.e.m. was calculated for all groups and compared by two-tailed paired Student’s t -test or by analysis of variance, with the Bonferroni multiple comparisons test for post hoc analysis. Unless otherwise stated, multiple comparisons were performed by analysis of variance. P <0.05 was used as the criteria for statistical significance. For Figs 1b and 4b , the Pearson product-moment correlation coefficient ( R 2 ) was calculated and a two-tailed P -value was generated from a probability table. Prism 3.0 software was used for all statistical analysis. How to cite this article: Lamoureux, F. et al . Selective inhibition of BET bromodomain epigenetic signalling interferes with the bone-associated tumour vicious cycle. Nat. Commun. 5:3511 doi: 10.1038/ncomms4511 (2014).